Functional characterization of the TERRA transcriptome at damaged telomeres Telomere deprotection occurs during tumorigenesis and aging upon telomere shortening or loss of the telomeric shelterin component TRF2. Deprotected telomeres undergo changes in chromatin structure and elicit a DNA damage response (DDR) that leads to cellular senescence. The telomeric long noncoding RNA TERRA has been implicated in modulating the structure and processing of deprotected telomeres. Here, we characterize the human TERRA transcriptome at normal and TRF2-depleted telomeres and demonstrate that TERRA upregulation is occurring upon depletion of TRF2 at all transcribed telomeres. TRF2 represses TERRA transcription through its homodimerization domain, which was previously shown to induce chromatin compaction and to prevent the early steps of DDR activation. We show that TERRA associates with SUV39H1 H3K9 histone methyltransferase, which promotes accumulation of H3K9me3 at damaged telomeres and end-to-end fusions. Altogether our data elucidate the TERRA landscape and defines critical roles for this RNA in the telomeric DNA damage response. The prevalent damage of the genetic material poses a particular threat to genome integrity and cell survival. Sensitivity of DNA to damaging agents and the kinetics of repair are influenced by the chromatin structure. The DNA damage response (DDR) differs in heterochromatic and euchromatic genomic loci. Heterochromatin is better protected from damage than euchromatin [1] but damaged heterochromatin is less accessible to DDR factors. Thus, DNA damage repair in heterochromatin occurs with slow kinetics and is less effective than in euchromatin, resulting in long-term retention of DNA lesions [2] . While the ataxia-telangiectasia mutated protein (ATM) prevents large-scale chromatin decompaction and silences transcription in cis next to DNA double strand breaks (DSBs) in euchromatic domains [3] , repair of damaged heterochromatic regions is likely to require decondensation of the surrounding chromatin structure and derepression of transcription [4] , [5] . Chromatin relaxation and subsequent repair of heterochromatin requires the ATM-dependent phosphorylation of the heterochromatin protein Kap-1 (ref. 6 ) and the rapid release of phosphorylated HP1 proteins from H3K9me3 (ref. 7 ), followed by association of Tip60, an acetyltransferase involved in chromatin acetylation [8] , [9] and in the modification and subsequent activation of ATM [10] , [11] , [12] . Telomeres resemble constitutive heterochromatin as they contain H3K9me3 and HP1 proteins [13] . Telomeres also actively repress DNA repair pathways to prevent recombination of natural chromosome ends. Consistent with these features, telomeres when damaged but still functional elicit a persistent DDR [14] and they are refractory to DNA repair [15] , thus causing cellular senescence [15] . In vertebrates, telomeric DNA is associated with specialized telomeric proteins, known as shelterins [16] , which repress DNA damage activation at the ends of linear chromosomes [17] . At functional telomeres, the shelterin component TRF2 binds double-stranded telomeric DNA and represses ATM signalling, whereas the single-stranded telomeric binding factor POT1 prevents ATR (ataxia telangiectasia and Rad3 related) activation [18] . Extensive telomere shortening leads to activation of the ATM and ATR pathways and replicative senescence which is thought to suppress tumorigenesis [19] , [20] , [21] , [22] . Telomeres in most or all eukaryotes are transcribed into heterogeneous long non-coding RNAs known as TERRA [23] , [24] . TERRA transcription is driven by RNA polymerase II (RNAPII) and proceeds from subtelomeric DNA into the telomeric repeat sequences [23] , [24] . In humans, CpG island promoters present at a subset of telomeres are partially responsible for driving TERRA transcription and PCR with reverse transcription (RT–PCR) analyses as well as FISH experiments suggested that several if not all telomeres can produce TERRA transcripts [25] . However, a comprehensive description of the whole TERRA transcriptome is missing. TERRA transcription has been linked to chromatin structure and is repressed by the DNA methyltransferase enzymes DNMT1 and DNMT3b [25] , [26] and by the SUV39H1 H3K9 histone methyltransferase and heterochromatin protein 1α (HP1α; ref. 27 ). TERRA partially colocalizes with telomeres [23] , [28] and it has been proposed that TERRA may contribute to telomeric heterochromatin formation by promoting H3K9 trimethylation [27] , [29] . Recently, we have shown that TERRA is bound by the lysine demethylase LSD1 at TRF2-depleted telomeres, which may promote the physical interaction between LSD1 and MRE11. LSD1 activates MRE11 for the nucleolytic processing of uncapped telomeres [28] . How TERRA transcription is regulated at dysfunctional telomeres and to what extent TERRA may affect chromatin reorganization following the induction of telomeric DDR remains to be elucidated. Here we characterize in detail the transcriptional upregulation of TERRA that ensues telomere deprotection upon depletion of TRF2. We find that TERRA upregulation is due to increased transcription of telomeres. It occurs independently of ATM-dependent checkpoint signalling and p53. We demonstrate that TRF2 negatively regulates TERRA transcription through its dimerization domain. We define the TERRA transcriptome and identify conserved transcription factor binding sites that may regulate TERRA transcription. Finally, we provide data supporting a model in which TERRA promotes SUV39H1 binding to TRF2-deficient telomeres and accumulation of H3K9me3. Thus, the increased density of H3K9me3 at uncapped telomeres may favour telomere end-to-end joining and the activation of Tip60 and the subsequent induction of the DDR pathways. TERRA levels increase upon DNA damage and TRF2 loss To investigate the putative impact of DNA damage on TERRA expression at human telomeres, we monitored TERRA levels in HeLa cells that had been continuously treated with the DSBs generating agent zeocin. FACS profile analysis of zeocin-treated cells showed an accumulation of cells in G2/M ( Supplementary Fig. 1a ), indicating a prolonged mitotic arrest upon persistent DNA damage. In chromatin immunoprecipitation (ChIP) experiments with antibodies against TRF2, less telomeric DNA was recovered upon zeocin treatment, indicating that reduced amounts of TRF2 remained associated with telomeres ( Fig. 1a,b ). At the same time ChIP analysis with antibodies against γ-H2AX indicated that this damage marker accumulated at telomeres ( Fig. 1c,d ). These results are in agreement with a previous report showing that prolonged mitotic arrest leads to loss of TRF2 from telomeres, telomere deprotection and DDR activation [30] . Next, we measured TERRA levels in time course experiments by northern blot analysis using a strand-specific TERRA probe. Quantification of the hybridization signals revealed that TERRA accumulated at late time points of zeocin treatment over 18S rRNA ( Fig. 1e ; Supplementary Fig. 1b ). To test whether TERRA upregulation was due to telomere deprotection and DDR activation, we monitored TERRA levels following shRNA-mediated depletion of TRF2 and POT1. As expected, shRNA-mediated depletion of TRF2 and POT1 in HeLa cells ( Supplementary Fig. 1a ) led to the accumulation of γ-H2AX at telomeric but not at centromeric regions as assessed by ChIP using antibodies against γ-H2AX ( Fig. 1f,g ). TERRA levels increased upon TRF2 knockdown but they remained unaltered in cells depleted of POT1 ( Fig. 1h ). Overall, our data suggest that TERRA accumulation upon persistent DNA damage involves depletion of TRF2 from telomeres. To evaluate whether other shelterin proteins may affect TERRA levels, analogous experiments were carried out in HeLa cells depleted for TRF1, Rap1, TIN2 and TPP1 ( Supplementary Fig. 2b ). As expected for a functional depletion of TRF1, TIN2 and TPP1, telomeric but not centromeric DNA was enriched in ChIP experiments using antibodies against γ-H2AX ( Supplementary Fig. 2c,d ). By northern blot analysis, we found that TERRA is also upregulated following TRF1 removal but not upon depletion of the other shelterin components ( Supplementary Fig. 2e ). 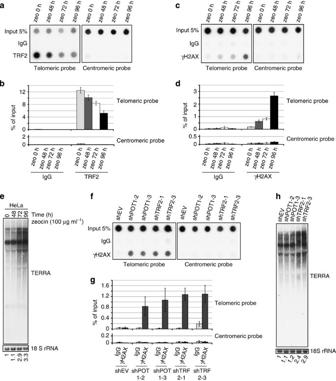Figure 1: TERRA expression is upregulated upon persistent DDR and TRF2 depletion. (a) DNA-ChIP of telomeric and centromeric DNA with anti-TRF2 antibody performed in HeLa cells treated with zeocin for the indicated times. (b) Quantification of three independent ChIP experiments represented ina(mean±s.d.,n=3). (c) DNA-ChIP of telomeric and centromeric DNA with anti-γH2AX antibody performed in HeLa cells treated with zeocin for the indicated times. (d) Quantification of three independent ChIP experiments represented inc(mean±s.d.,n=3). (e) Northern blot analysis of total RNA from HeLa cells treated with zeocin. TERRA was detected using a telomeric DNA probe complementary to the UUAGGG repeats. Filters were then stripped and reprobed for 18S rRNA. (f) DNA-ChIP of telomeric and centromeric DNA with anti-γH2AX antibody performed in HeLa cells depleted of POT1 and TRF2, respectively. (g) Quantification of three independent ChIP experiments represented inf(mean±s.d.,n=3). (h) Northern blot analysis of total RNA from HeLa cells depleted of POT1 and TRF2. Figure 1: TERRA expression is upregulated upon persistent DDR and TRF2 depletion. ( a ) DNA-ChIP of telomeric and centromeric DNA with anti-TRF2 antibody performed in HeLa cells treated with zeocin for the indicated times. ( b ) Quantification of three independent ChIP experiments represented in a (mean±s.d., n =3). ( c ) DNA-ChIP of telomeric and centromeric DNA with anti-γH2AX antibody performed in HeLa cells treated with zeocin for the indicated times. ( d ) Quantification of three independent ChIP experiments represented in c (mean±s.d., n =3). ( e ) Northern blot analysis of total RNA from HeLa cells treated with zeocin. TERRA was detected using a telomeric DNA probe complementary to the UUAGGG repeats. Filters were then stripped and reprobed for 18S rRNA. ( f ) DNA-ChIP of telomeric and centromeric DNA with anti-γH2AX antibody performed in HeLa cells depleted of POT1 and TRF2, respectively. ( g ) Quantification of three independent ChIP experiments represented in f (mean±s.d., n =3). ( h ) Northern blot analysis of total RNA from HeLa cells depleted of POT1 and TRF2. Full size image TERRA transcriptome analysis at TRF2-deprotected telomeres TERRA transcription initiates within subtelomeric regions and proceeds into the telomeric TTAGGG-tracts. TERRA promoters have been identified within CpG islands that are embedded within repetitive DNA tracts referred to as 61-29-37 repeats [25] . These subtelomeric repeats reside in close proximity of the telomeric TTAGGG-repeats at a large number of chromosome ends [25] . To comprehensively characterize the TERRA transcriptome, we performed high-throughput sequencing using nuclear RNA from wild-type and TRF2-depleted HeLa cells. To enrich for full-length TERRA and minimize ribosomal RNA (rRNA) contamination, we used two purification steps. Since TERRA, but not rRNAs, contains a canonical m7G cap [28] , nuclear RNA was first incubated with the high-affinity m7G cap-binding protein eIF4E fused to GST and immobilized on Glutathione-Sepharose. The RNA was recovered from the beads and incubated with biotinylated antisense (CCCTAA) 3 oligonucleotides that specifically annealed to the UUAGGG-tracts residing near the 3′ends of TERRA transcripts. The RNA bound to biotinylated antisense (CCCTAA) 3 oligonucleotides was recovered from streptavidin beads. RNA-seq experiments were performed on the TERRA-enriched RNA fraction and on total nuclear RNA (input) from wild-type or TRF2-depleted HeLa cells. The reads were mapped to the most complete assembly available of human subtelomeres ( http://www.wistar.org/lab/harold-c-riethman-phd/page/subtelomere-assemblies ) [31] and read density profiles were generated counting the number of reads aligned at each position along the subtelomeric regions. The TERRA transcripts stemming from different chromosome ends were identified based on their enriched read density in the UUAGGG-containing RNA fraction compared with the input material. Doing so, we identified 10 distinct chromosome ends where transcription into TERRA molecules started as far as 5–10 kb upstream of the subtelomere–telomere boundary (see Fig. 2a for TRF2-depleted HeLa cells and Supplementary Fig. 3 for wild-type HeLa cells). At eight other chromosome ends, the RNA-seq data suggested that transcription starts in close proximity to the TTAGGG-tracts ( Supplementary Fig. 4 ). Despite good mappability scores for several additional chromosome ends, the remaining complete subtelomeres did not display consistent read profiles in the subtelomeric regions ( Supplementary Fig. 5 ). However, due to the repetitive nature of the human telomeric repeat sequences, the reads containing only UUAGGG repeats could not be assigned to a specific chromosome end. Thus, we cannot rule out that transcription at several chromosome termini may initiate within the terminal TTAGGG-repeat sequences. Our RNA-seq data also revealed that TERRA 5′ ends are embedded within subtelomeric regions with higher GC content than the non-transcribed subtelomeres ( Fig. 2b ). In addition, using published ChIP-seq data from Deng et al. [32] , we ascertain that CTCF, which positively regulates TERRA transcription, binds subtelomeres in the vicinity of TERRA 5′ ends ( Fig. 2a ; Supplementary Fig. 4 ). 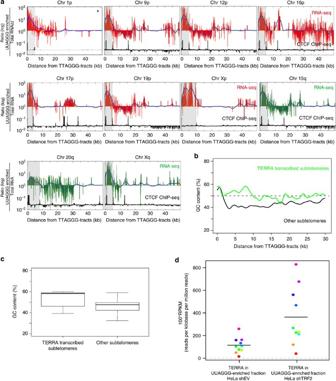Figure 2: Characterization of TERRA transcriptome at TRF2-depleted telomeres. (a) Enrichment profiles of RNA-seq data of UUAGGG-containing RNAs versus total nuclear RNA prepared from HeLa cells depleted of TRF2 at 10 different chromosome ends showing transcription within subtelomeric regions. Red and green labelling indicates the p- and the q-arms, respectively. Yellow rectangles indicate TTAGGG repeats interspersed in subtelomeric regions. The blue line is a moving average over a window of 10 nucleotides. Enrichment profiles of ChIP-seq analysis of CTCF are shown below the RNA-seq profile data for each chromosome end. (b) Comparison of the GC content of TERRA transcribed versus non-transcribed subtelomeres. The plots were generated using the Wistar GC content track and are an average of the two subtelomere subsets. (c) Average GC content calculated in the first 5 kb of each subtelomere. The boxes represent the GC content distribution of the two subtelomere subsets (TERRA transcribed versus non-transcribed subtelomeres). The middle line is the median, whereas the lower and upper bounds are the mininimal and maximal values. (d) Reads per kilobase per million reads (RPKM, times 102for practicality) as a measure for chromosome-specific TERRA levels in wild-type (shEV) and TRF2-depleted cells (shTRF2). Figure 2: Characterization of TERRA transcriptome at TRF2-depleted telomeres. ( a ) Enrichment profiles of RNA-seq data of UUAGGG-containing RNAs versus total nuclear RNA prepared from HeLa cells depleted of TRF2 at 10 different chromosome ends showing transcription within subtelomeric regions. Red and green labelling indicates the p- and the q-arms, respectively. Yellow rectangles indicate TTAGGG repeats interspersed in subtelomeric regions. The blue line is a moving average over a window of 10 nucleotides. Enrichment profiles of ChIP-seq analysis of CTCF are shown below the RNA-seq profile data for each chromosome end. ( b ) Comparison of the GC content of TERRA transcribed versus non-transcribed subtelomeres. The plots were generated using the Wistar GC content track and are an average of the two subtelomere subsets. ( c ) Average GC content calculated in the first 5 kb of each subtelomere. The boxes represent the GC content distribution of the two subtelomere subsets (TERRA transcribed versus non-transcribed subtelomeres). The middle line is the median, whereas the lower and upper bounds are the mininimal and maximal values. ( d ) Reads per kilobase per million reads (RPKM, times 10 2 for practicality) as a measure for chromosome-specific TERRA levels in wild-type (shEV) and TRF2-depleted cells (shTRF2). Full size image Next, we identified cis- regulatory elements and transcription factors (TFs) that may control TERRA expression. To this aim, we used TRANSFAC databases and scanned for transcriptional regulatory modules in the subtelomeric regions flanking the identified TERRA transcription start sites. For the TERRA promoters located 5–10 kb upstream of the telomeric tracts, our analysis revealed an overrepresentation of binding sites for zinc finger transcription factors (ZFP281, ZFP740 and ZFX) and members of the SP/KLF (specificity protein/Kruppel-like factor) family, such as KLF15, SP1, SP2 and SP4 ( Supplementary Table 1 ). On the other hand, the TERRA promoters located in close proximity of the terminal TTAGGG-repeat sequences displayed an overrepresentation of sequence motifs that can be bound by interferon regulatory factors, basic helix-loop-helix transcription factors, such as myogenic regulatory factors (MyoD, Myf, Myogenin) and GATA-type zinc finger transcription factors (GATA1 and GATA5) ( Supplementary Table 2 ). The binding motif for the transcriptional factor CTCF is overrepresented at both the telomere distal and proximal TERRA promoters ( Supplementary Tables 1 and 2 ), thus further supporting the role of CTCF in regulating TERRA expression. 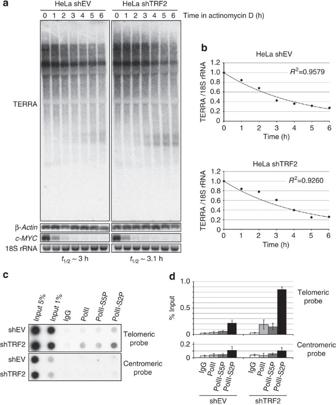Figure 3: TERRA transcriptional rate but not half-life increases upon TRF2 depletion. (a) TERRA half-life. Wild-type and TRF2-depleted HeLa cells were treated with 5 μg ml−1actinomycin D for the indicated times. Total RNA was prepared and subjected to Northern blot analysis using a telomeric DNA probe detecting UUAGGG repeats. Filters were then stripped and reprobed successively for c-MYC, β-actin and 18S rRNA. (b) Quantification of TERRA half-life in wild-type and TRF2-depleted HeLa cells based on northern blots shown ina. Relative TERRA levels were calculated using a scatter plot analysis after normalizing TERRA to 18S rRNA. The best-fit exponential regression curve of the data points was determined for both conditions.R2values are indicated. (c) DNA-ChIP of telomeric and centromeric DNA with anti-RNAPII antibodies performed in HeLa cells depleted of TRF2. (d) Quantification of three independent ChIP experiments represented inc(mean±s.d.,n=3). Finally, we compared the abundance of the different TERRA molecules that contained long subtelomeric sequences by calculating the number of reads per kilobase per million reads (RPKM) [33] in the region between the TERRA 5′ ends and the start of the telomeric tract (5–10 kb; not spliced; Supplementary Table 3 ). The abundance of TERRA RNAs from the different chromosome ends was in the same bulk part and TERRA abundance increased similarly at all measured chromosome ends 2 to 4-fold upon depletion of TRF2 confirming the previous results ( Fig. 2d and Supplementary Table 3 ). The TERRA RPKMs were compared with the values obtained for four different housekeeping genes. TERRA abundance from individual chromosomes ends was 10 times lower than transcripts from the GUSB gene (encoding for β-glucuronidase) and 100 to 1,000 times lower than the transcripts of three other highly expressed housekeeping genes ( GAPDH , ACTB and TUBA1 ) ( Supplementary Table 3 ). Increased transcription in TRF2-deficient cells TERRA upregulation at deprotected telomeres could be a result of a longer half-life of the transcripts or an increased transcription rate. To distinguish between these two possibilities, we first measured TERRA half-life. We blocked transcription in wild-type and TRF2-depleted HeLa cells with actinomycin D and monitored TERRA levels in time course experiment by northern blot analysis. β-Actin, c-Myc and 18S rRNA were included in the analysis for normalization (β-actin and 18S rRNA) and to control for successful inhibition of RNAPII (c-Myc) (( t1/2 ) of 20 min (refs 34 , 35 , 36 ); Fig. 3a ). Quantification of the hybridization signals revealed that, as previously shown [23] , [28] , total TERRA has a half-life of ~3 h in wild-type cells. In TRF2-depleted cells, the half-life increased only marginally to ~3.1 h upon TRF2 removal ( Fig. 3b ), which cannot account for the accumulation of TERRA transcripts in TRF2-deficient cells. Figure 3: TERRA transcriptional rate but not half-life increases upon TRF2 depletion. ( a ) TERRA half-life. Wild-type and TRF2-depleted HeLa cells were treated with 5 μg ml −1 actinomycin D for the indicated times. Total RNA was prepared and subjected to Northern blot analysis using a telomeric DNA probe detecting UUAGGG repeats. Filters were then stripped and reprobed successively for c-MYC, β-actin and 18S rRNA. ( b ) Quantification of TERRA half-life in wild-type and TRF2-depleted HeLa cells based on northern blots shown in a . Relative TERRA levels were calculated using a scatter plot analysis after normalizing TERRA to 18S rRNA. The best-fit exponential regression curve of the data points was determined for both conditions. R 2 values are indicated. ( c ) DNA-ChIP of telomeric and centromeric DNA with anti-RNAPII antibodies performed in HeLa cells depleted of TRF2. ( d ) Quantification of three independent ChIP experiments represented in c (mean±s.d., n =3). Full size image To obtain clues about transcriptional activity at wild-type and TRF2-depleted telomeres, we performed ChIP experiments using antibodies against RNA polymerase II (RNAPII) and its phosphorylated forms ( Fig. 3c,d ). Telomeric DNA was significantly enriched in TRF2-depleted cells over wild-type cells with all RNAPII antibodies. Most striking was the difference with an antibody against the elongating form of RNAPII recognizing the phosphorylated serine in the amino acid 2 position of the YSPTSPS-repeat sequence in the carboxy (C)-terminal domain of RNAPII (PolII-S2P in Fig. 3c,d ). Together, these experiments indicate that TERRA accumulation upon telomere deprotection is not because of an increase in the stability of the transcript but is caused by a higher transcription rate. Damage signalling is not required for TERRA upregulation To assess the influence of DNA damage signalling on the increased levels of TERRA upon TRF2 knockdown, we depleted separately MRE11 or NBS1, two subunits of the MRN complex, and the ATM and ATR kinases by shRNA. MRE11 or NBS1 were efficiently depleted in wild-type and TRF2-deficient HeLa cells as determined by western blot analyses ( Fig. 4a ). Furthermore, a reduction of telomere end-to-end fusions in the TRF2-depleted cells indicated loss of function of MRE11 and NBS1 ( Supplementary Fig. 6a ). TERRA levels were monitored by northern blot analysis and quantitative RT–PCR. Depletion of the MRN complex components neither affected TERRA levels in wild-type cells nor did it prevent TERRA upregulation at TRF2-deprotected telomeres ( Fig. 4b ; Supplementary Fig. 6e ). Similar experiments were performed in wild-type and TRF2-deficient cells efficiently depleted of ATM and ATR ( Fig. 4c ). The depletions of ATM and ATR both were functional as phosphorylation of the downstream Chk2 and Chk1 kinases was reduced ( Supplementary Fig. 6b ). Functional depletion of ATM was further confirmed in ChIP experiments in which γ-H2AX no longer accumulated at telomeres in TRF2-deficient cells ( Supplementary Fig. 6c,d ). Analogous to what was observed for the MRN complex, depletion of ATM and ATR had no effect on TERRA levels at both functional and deprotected telomeres ( Fig. 4d ; Supplementary Fig. 6f ). In addition to ATM and ATR, we depleted SMG1, which is also a member of the PI3K-related kinase (PIKK) family. SMG1 has well-characterized roles in nonsense-mediated RNA decay and in the DDR [37] , [38] . In addition, SMG1 negatively regulates the abundance of TERRA at telomeres [23] . We knocked down SMG1 with two different shRNAs alone or in combination with TRF2 ( Supplementary Fig. 7a ), which concomitantly reduced phosphorylation of UPF1 as expected for loss function of SMG1 ( Supplementary Fig. 7b ) and evaluated TERRA levels by quantitative RT–PCR. No significant difference in TERRA levels was observed upon SMG1 depletion in both wild-type and TRF2-deficient cells ( Supplementary Fig. 7c ). Finally, we tested if p53 may control TERRA induction upon telomere deprotection. For this, we employed two isogenic human colorectal carcinoma cell lines (HCT116), which were wild-type (p53+/+) or knocked out for p53 (p53 −/− ; ref. 39 ). We transfected the p53 +/+ and the p53 −/− cells with shRNAs against POT1 or TRF2 and we found that TERRA upregulation occurred upon TRF2 but not POT1 removal in presence and absence of p53 ( Fig. 4e ). Thus p53 is dispensable for TERRA transcription at wild-type and TRF2-deprotected telomeres. Overall, these results strongly suggest that DDR activation does not account for TERRA upregulation following telomere deprotection by TRF2. Therefore, we postulated that TRF2 might act directly as a negative regulator of TERRA transcription. 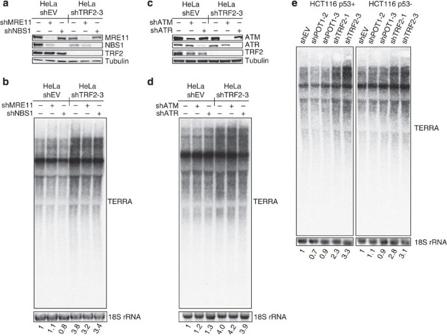Figure 4: DDR activation is not required for TERRA upregulation at uncapped telomeres. (a) Western blot analysis to evaluate knockdown efficiency of endogenous MRE11, NBS1 and TRF2. Tubulin was used as loading control. (b) Wild-type (shEV) and TRF2-depleted (shTRF2) HeLa cells transfected with control vector (shEV) or additionally depleted for MRE11 (shMRE11) and NBS1 (shNBS1). Total RNA was prepared and subjected to northern blot analysis using a telomeric DNA probe detecting UUAGGG repeats. Filters were then stripped and reprobed subsequently for 18S rRNA. (c) Western blot analysis to evaluate knockdown efficiency of endogenous ATM, ATR and TRF2. Tubulin was used as loading control. (d) Wild-type (shEV) and TRF2-deficient (shTRF2) HeLa cells transfected with control vector (shEV) or depleted for ATM (shATM) and ATR (shATR). Total RNA was prepared and subjected to northern blot analysis using a telomeric DNA probe detecting UUAGGG repeats. Filters were then stripped and reprobed subsequently for 18S rRNA. (e) Northern blot analysis of total RNA prepared wild-type (p53+) and p53 knockout (p53−) HCT116 cells. The blot was probed using a telomeric DNA probe detecting UUAGGG repeats. The filter was stripped and reprobed subsequently for 18S rRNA. Uncropped western blots are shown inSupplementary Fig. 9a,b. Figure 4: DDR activation is not required for TERRA upregulation at uncapped telomeres. ( a ) Western blot analysis to evaluate knockdown efficiency of endogenous MRE11, NBS1 and TRF2. Tubulin was used as loading control. ( b ) Wild-type (shEV) and TRF2-depleted (shTRF2) HeLa cells transfected with control vector (shEV) or additionally depleted for MRE11 (shMRE11) and NBS1 (shNBS1). Total RNA was prepared and subjected to northern blot analysis using a telomeric DNA probe detecting UUAGGG repeats. Filters were then stripped and reprobed subsequently for 18S rRNA. ( c ) Western blot analysis to evaluate knockdown efficiency of endogenous ATM, ATR and TRF2. Tubulin was used as loading control. ( d ) Wild-type (shEV) and TRF2-deficient (shTRF2) HeLa cells transfected with control vector (shEV) or depleted for ATM (shATM) and ATR (shATR). Total RNA was prepared and subjected to northern blot analysis using a telomeric DNA probe detecting UUAGGG repeats. Filters were then stripped and reprobed subsequently for 18S rRNA. ( e ) Northern blot analysis of total RNA prepared wild-type (p53+) and p53 knockout (p53−) HCT116 cells. The blot was probed using a telomeric DNA probe detecting UUAGGG repeats. The filter was stripped and reprobed subsequently for 18S rRNA. Uncropped western blots are shown in Supplementary Fig. 9a,b . Full size image The homodimerization domain of TRF2 represses TERRA TRF2 and TRF1 both consist of four domains: a C-terminal MYB domain required for binding to telomeres, a flexible hinge domain involved in protein–protein interactions, a TRFH domain required for homodimerization [40] and chromatin compaction [41] , [42] , and a divergent amino (N)-terminal region rich in basic amino acids in TRF2 and acidic residues in TRF1. To identify the molecular properties of TRF2 involved in regulating TERRA transcription, we swapped, inspired by a previous study [41] , several domains between TRF2 and TRF1 (refs 43 , 44 ) in cDNA constructs ( Fig. 5a ) and expressed them in HeLa cells ( Fig. 5b ). Western blot analysis and IF-FISH experiments indicated that the TRF2/TRF1 chimeric proteins were expressed at comparable levels ( Fig. 5b ) and that they localized to telomeres even though the nucleoplasmic patterns differed slightly with the different constructs ( Fig. 5c ). We then tested whether the TRF2 chimeric constructs were able to prevent induction of TERRA transcription in HeLa cell lines depleted of endogenous TRF2 by shRNA. Importantly, ectopically expressed full-length wild-type TRF2 but not TRF1 prevented TERRA upregulation upon depletion of endogenous TRF2 ( Fig. 5d ). This suggests that TRF2 and TRF1 suppress TERRA abundance through distinct mechanisms. The TRF2 construct lacking the N-terminal basic region (TRF2-ΔB) was also able to suppress the transcriptional induction of TERRA that followed loss of endogenous TRF2 ( Fig. 5d ) ruling out a critical and specific function of this domain in TRF2. Similarly, the hinge and DNA binding domains of TRF2 also did not seem to have critical roles for the TRF2-specific repression of TERRA as they could be replaced with the corresponding domains from TRF1 (TRF2-ΔBcH and TRF2-ΔBcM in Fig. 5 ). In contrast, ectopic expression of the TRF2 chimeric protein containing the TRFH domain of TRF1 (TRF2-ΔBcT) did not prevent TERRA accumulation in the absence of endogenous TRF2 ( Fig. 5d ). Overall, these data suggest that TRF2 represses TERRA transcription through its TRFH domain. This domain may elicit this function through its capacity in structural compaction of chromatin [41] , [42] , making telomeres less accessible to RNAPII. Interestingly, it has recently been shown that the TRFH domain of TRF2 is also required to prevent the activation of the ATM pathway and the initial steps in the telomeric DDR [44] . 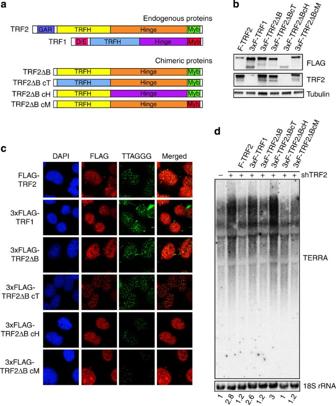Figure 5: TRF2 negatively regulates TERRA transcription through its homodimerization TRFH domain. (a) Schematic representation of TRF2/TRF1 chimeric constructs. (b) Western blot analysis to test expression of TRF2/TRF1 chimeric proteins in HeLa cells depleted of endogenous TRF2. Uncropped blots are shown inSupplementary Fig. 9c. (c) Immunofluorescence fluorescencein situhybridization (IF-FISH) analysis to assess the localization of the TRF2/TRF1 chimeric proteins (red signals) at telomeres (green signals) in HeLa cells depleted of endogenous TRF2. (d) Northern blot analysis. Total RNA was prepared from wild-type HeLa cells or HeLa cells depleted of TRF2 that had been transfected with the indicated constructs. Northern blot analysis was then performed using a telomeric DNA probe detecting UUAGGG repeats. Filters were then stripped and reprobed subsequently for 18S rRNA. Figure 5: TRF2 negatively regulates TERRA transcription through its homodimerization TRFH domain. ( a ) Schematic representation of TRF2/TRF1 chimeric constructs. ( b ) Western blot analysis to test expression of TRF2/TRF1 chimeric proteins in HeLa cells depleted of endogenous TRF2. Uncropped blots are shown in Supplementary Fig. 9c . ( c ) Immunofluorescence fluorescence in situ hybridization (IF-FISH) analysis to assess the localization of the TRF2/TRF1 chimeric proteins (red signals) at telomeres (green signals) in HeLa cells depleted of endogenous TRF2. ( d ) Northern blot analysis. Total RNA was prepared from wild-type HeLa cells or HeLa cells depleted of TRF2 that had been transfected with the indicated constructs. Northern blot analysis was then performed using a telomeric DNA probe detecting UUAGGG repeats. Filters were then stripped and reprobed subsequently for 18S rRNA. Full size image TERRA upregulation may sustain H3K9me3 accumulation At telomeres, it has been suggested that TERRA may participate in the accumulation of H3K9me3 (refs 27 , 29 ). We investigated by ChIP the histone methylation pattern upon telomere uncapping. The density of monomethylated H3K4 was not affected following TRF2 depletion and the signals for di- and trimethylated H3K4 were close to background at both, capped and unprotected telomeres ( Supplementary Fig. 8a,b ). Also monomethyl H3K9 was not affected at telomeres following TRF2 depletion ( Fig. 6a ). However, we observed a significant reduction of dimethylated H3K9 (H3K9me2) and a corresponding rise in the density of H3K9me3 upon telomere uncapping, whereas they both remained unaltered at centromeric chromatin ( Fig. 6a,b ). At DSBs occurring in heterochromatic regions, H3K9me3 provides activation sites for Tip60 (KAT5) (ref. 10 ), which affects H4K16 acetylation and ATM activation. In line with this, we observed that TRF2-deprotected telomeres showed an increase in H4K16 acetylation, which is indicative of Tip60 activity ( Supplementary Fig. 8c ). We tested whether the accumulation of H3K9me3 at dysfunctional telomeres coincides with recruitment of the histone methyltransferase SUV39H1. We performed ChIP experiments with two different antibodies against endogenous SUV39H1 and found that the telomeric signal in the SUV39H1-ChIP significantly increased upon telomere uncapping by TRF2 depletion ( Fig. 6c,d ) suggesting that this protein is responsible for H3K9 trimethylation at TRF2-depleted telomeres. Next, we assessed whether SUV39H1 can interact with TERRA. To this aim, we performed RNA immunoprecipitation experiments with extracts derived from formaldehyde-crosslinked HeLa cells followed by stringent washing conditions. Approximately 1% of TERRA was immunoprecipitated with two different antibodies against endogenous SUV39H1 upon telomere uncapping. In contrast, this interaction was barely detectable in cells with normal levels of TRF2. Thus the number of TERRA–SUV39H1 complexes increased substantially upon TRF2 removal ( Fig. 6e ). Remarkably, TERRA was also significantly enriched upon H3K9me3 RNA-IP of formaldehyde-crosslinked extracts following telomere deprotection indicating that TERRA, SUVH39H1 and H3K9me3 may be present in common structures. The specificity of these interactions was confirmed by the fact that TERRA did not immunoprecipitate with IgG control. 18S rRNA served as negative control and was not retrieved by SUV39H1 or H3K9me3 immunoprecipitation. Together, these experiments indicate that TERRA upregulation may account for the increased recruitment of SUV39H1 to uncapped telomeres and the subsequent accumulation of H3K9me3 upon depletion of TRF2. 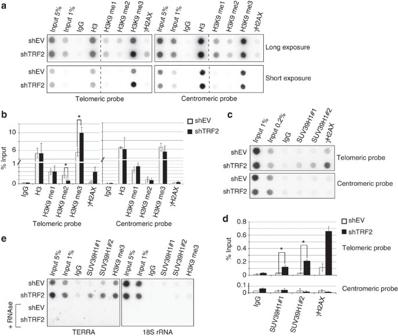Figure 6: SUV39H1 associates with TERRA and is recruited to uncapped telomeres. (a) ChIP of telomeric and centromeric DNA with H3 antibodies recognizing histone marks in HeLa cells transfected with control vector (shEV) or depleted of TRF2 (shTRF2). (b) Quantification of three independent ChIP experiments represented ina(mean±s.d.,n=3). Statistical analysis was done using a two-tailed Student’st-test (*P<0.05). (c) ChIP of telomeric and centromeric DNA with anti-SUV39H1 antibodies performed in HeLa cells transfected with control vector (shEV) or depleted of TRF2 (shTRF2). (d) Quantification of three different ChIP experiments represented inc(mean±s.d.,n=3). Statistical analysis was done using a two-tailed Student’st-test (*P<0.05). (e) RNA-ChIP assays with two antibodies against endogenous SUV39H1 performed in HeLa cells transfected with control vector (shEV) or depleted of TRF2 (shTRF2). IP-recovered RNA was detected with probes annealing with TERRA (left panel) or 18S rRNA (right panel). Figure 6: SUV39H1 associates with TERRA and is recruited to uncapped telomeres. ( a ) ChIP of telomeric and centromeric DNA with H3 antibodies recognizing histone marks in HeLa cells transfected with control vector (shEV) or depleted of TRF2 (shTRF2). ( b ) Quantification of three independent ChIP experiments represented in a (mean±s.d., n =3). Statistical analysis was done using a two-tailed Student’s t -test (* P <0.05). ( c ) ChIP of telomeric and centromeric DNA with anti-SUV39H1 antibodies performed in HeLa cells transfected with control vector (shEV) or depleted of TRF2 (shTRF2). ( d ) Quantification of three different ChIP experiments represented in c (mean±s.d., n =3). Statistical analysis was done using a two-tailed Student’s t -test (* P <0.05). ( e ) RNA-ChIP assays with two antibodies against endogenous SUV39H1 performed in HeLa cells transfected with control vector (shEV) or depleted of TRF2 (shTRF2). IP-recovered RNA was detected with probes annealing with TERRA (left panel) or 18S rRNA (right panel). Full size image SUV39H1 N-terminus binds the UUAGGG repeats of TERRA To assess whether SUV39H1 binds TERRA directly, the biochemical properties of recombinant GST-SUV39H1 were characterized in electromobility shift assays (EMSAs). GST-SUV39H1 was expressed in E. coli , purified ( Fig. 7a ) and incubated with labelled TERRA-mimicking RNA oligonucleotide (UUAGGG) 10 . The affinity of purified SUV39H1 for TERRA-mimicking RNA oligonucleotides was shown by the retarded migration of the labelled oligonucleotide ( Fig. 7b ) and the identity of the shifted complex was confirmed in supershift mobility assays with the use of an antibody recognizing GST-SUV39H1 ( Fig. 7c ). In contrast to the TERRA-oligonucleotide, labelled DNA of the same sequence (TTAGGG) 10 was not bound by SUV39H1 ( Fig. 7b ). Further, the binding specificity was addressed by EMSA in competition experiments in which the association to labelled (UUAGGG) 7 -TERRA repeats was challenged with excess of unlabelled wild-type and mutant telomeric repeats ( Fig. 7d ). This analysis indicated that SUV39H1 has specificity for the AGGG sequence within the UUAGGG-repeats but it does not recognize the UU-dinucleotide ( Fig. 7d ). Finally, we delineated the TERRA interaction domains of SUV39H1. Two bacterially expressed GST-SUV39H1 fragments were purified ( Fig. 7e,f ) and characterized by EMSA for their ability to bind TERRA-mimicking RNA oligonucleotides (UUAGGG) 10 . Only the N-terminal SUV39H1 fragment encompassing the chromodomain was able to substantially retard the migration of the labelled TERRA-mimicking oligonucleotide ( Fig. 7g ) with a dissociation constant for (UUAGGG) 10 of ~80 nM. In summary, we conclude that SUV39H1 can bind directly via its N-terminal chromodomain the UUAGGG-repeat array of the TERRA transcript, with moderate specificity. 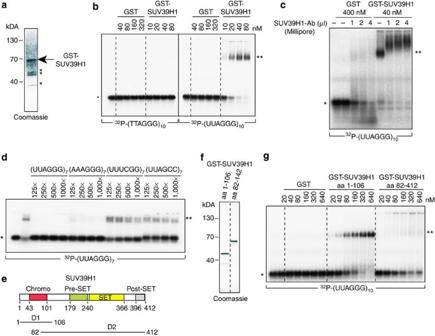Figure 7: The N-terminal domain of SUV39H1 directly binds UUAGGG-TERRA repeats. (a) Coomassie stained gel of GST-SUV39H1 affinity purified fromE. coli. Bands labelled with asterisks are SUV39H1 degradation products. (b) Agarose EMSA used to measure SUV39H1 RNA binding activityin vitro. GST-SUV39H1 was assayed for binding to32P-(UUAGGG)10RNA or32P-(TTAGGG)10DNA oligonucleotides, respectively. Single asterisks indicate free oligonucleotides and double asterisks protein/oligonucleotide complexes. (c) Agarose supershift assay performed with GST-SUV39H1 incubated with32P-(UUAGGG)10RNA oligonucleotide and an antibody recognizing SUV39H1 polypeptide. Single asterisks indicate free oligonucleotides and double asterisks protein/oligonucleotide complexes. (d) EMSA competition experiments of GST-SUV39H1 binding to32P-(UUAGGG)7. Increasing amounts of unlabeled (UUAGGG)7, (AAAGGG)7, (UUUCGG)7and (UUAGCC)7RNA oligonucleotides were added as competitors. Numbers indicate fold excess of competitor over32P-labelled probe. Single asterisks indicate free oligonucleotides and double asterisks protein/oligonucleotide complexes. (e) Scheme of SUV39H1 domains and deletion constructs. (f) Coomassie stained gel of GST-SUV39H1 deletion constructs affinity purified fromE. coli. (g) Agarose EMSA used to identify domains of SUV39H1 with binding activity for32P-(UUAGGG)10RNA oligonucleotides. Single asterisks indicate free oligonucleotides and double asterisks protein/oligonucleotide complexes. Figure 7: The N-terminal domain of SUV39H1 directly binds UUAGGG-TERRA repeats. ( a ) Coomassie stained gel of GST-SUV39H1 affinity purified from E. coli . Bands labelled with asterisks are SUV39H1 degradation products. ( b ) Agarose EMSA used to measure SUV39H1 RNA binding activity in vitro . GST-SUV39H1 was assayed for binding to 32 P-(UUAGGG) 10 RNA or 32 P-(TTAGGG) 10 DNA oligonucleotides, respectively. Single asterisks indicate free oligonucleotides and double asterisks protein/oligonucleotide complexes. ( c ) Agarose supershift assay performed with GST-SUV39H1 incubated with 32 P-(UUAGGG) 10 RNA oligonucleotide and an antibody recognizing SUV39H1 polypeptide. Single asterisks indicate free oligonucleotides and double asterisks protein/oligonucleotide complexes. ( d ) EMSA competition experiments of GST-SUV39H1 binding to 32 P-(UUAGGG) 7 . Increasing amounts of unlabeled (UUAGGG) 7 , (AAAGGG) 7 , (UUUCGG) 7 and (UUAGCC) 7 RNA oligonucleotides were added as competitors. Numbers indicate fold excess of competitor over 32 P-labelled probe. Single asterisks indicate free oligonucleotides and double asterisks protein/oligonucleotide complexes. ( e ) Scheme of SUV39H1 domains and deletion constructs. ( f ) Coomassie stained gel of GST-SUV39H1 deletion constructs affinity purified from E. coli . ( g ) Agarose EMSA used to identify domains of SUV39H1 with binding activity for 32 P-(UUAGGG) 10 RNA oligonucleotides. Single asterisks indicate free oligonucleotides and double asterisks protein/oligonucleotide complexes. Full size image To assess the roles of SUV39H1 in telomere end-to-end fusions at TRF2-depleted telomeres, we used a HeLa cell line in which TRF2 can be depleted by doxycycline-inducible expression of shRNAs [45] ( Fig. 8a ). Significantly, depletion of SUV39H1 by siRNAs in the TRF2-depleted cell line ( Fig. 8b ) reduced telomere end-to-end fusion events ( Fig. 8c and Supplementary Table 4 ) indicating that the chromatin modifications induced by this enzyme sustain end-to-end fusions in accordance with data obtained in mouse cells upon deletion of SUV39H1 (ref. 46 ). 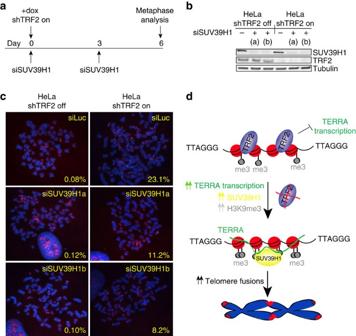Figure 8: SUV39H1 sustains telomere end fusions occurring upon TRF2 depletion. (a) Timeline of the experiment inbandc). (b) Western blot of total protein extracts from HeLa cells with or without shTRF2 expression and siRNAs transfection. Uncropped blots are shown inSupplementary Fig. 9d. (c) Metaphase chromosome spreads and telomere-FISH performed on HeLa cells depleted (shTRF2 on) or not depleted (shTRF2 off) for TRF2 and concomitantly transfected with siRNAs against luciferase (siLuc) or SUV39H1 (siSUV39H1a and siSUV39H1b). (d) Model for the regulation and here-described roles of TERRA at dysfunctional telomeres. Figure 8: SUV39H1 sustains telomere end fusions occurring upon TRF2 depletion. ( a ) Timeline of the experiment in b and c ). ( b ) Western blot of total protein extracts from HeLa cells with or without shTRF2 expression and siRNAs transfection. Uncropped blots are shown in Supplementary Fig. 9d . ( c ) Metaphase chromosome spreads and telomere-FISH performed on HeLa cells depleted (shTRF2 on) or not depleted (shTRF2 off) for TRF2 and concomitantly transfected with siRNAs against luciferase (siLuc) or SUV39H1 (siSUV39H1a and siSUV39H1b). ( d ) Model for the regulation and here-described roles of TERRA at dysfunctional telomeres. Full size image In this study, we characterize the transcriptional response of telomeres that follows uncapping upon depletion of TRF2. Our data show that damaged telomeres are transcriptionally derepressed which is typical for damaged heterochromatic domains. Using high-throughput RNA-seq, we also characterize the whole TERRA transcriptome. Our results demonstrate that transcription initiation of TERRA at different chromosome ends varies substantially with regard to its position to the telomeric repeat tract extending in some cases for several kilobases into the subtelomeric regions. This observation is in agreement with a broad distribution of RNAPII across subtelomeres that was reported previously [32] . Analysis of the subtelomeric sequence reads did not reveal any splicing events of TERRA transcripts suggesting that TERRA transcripts in contrast to many other long noncoding RNAs are not spliced. Sequences with enriched GC content located from 5–10 kb upstream of the telomeric tracts may function as promoters and drive TERRA transcription near at least 10 different chromosome ends. On the other hand, the previously reported set of CpG island promoters [25] appear responsible for driving the transcription of the TERRA molecules whose 5′ ends localize in close proximity to the telomeric tracts. Overall, the promoter distribution of TERRA at different chromosome ends can account for the length heterogeneity of the transcripts. We cannot rule out the possibility that transcription may also start within telomeric repeats or within immediate proximity thereof, leading us to underestimate the real number of transcribed chromosome ends; similarly, we cannot rule out cell line-specific effects that could impact the distribution of TERRA-expressing telomeres. We provide a bioinformatic analysis of the putative TERRA promoters and identify transcription factor modules that might regulate TERRA. Among the putative TERRA transcription factors, we find that CTCF, previously shown to regulate TERRA expression [32] , not only localizes near the 5′ ends of the CpG island TERRA promoters but also to the more telomere distal TERRA promoters identified in our analysis. Despite a previous study that reported a p53-dependent increase in TERRA levels at damaged telomeres [47] , we provide evidence that TERRA induction at TRF2-depleted telomeres occurs independently of p53 and does not require the ATM- or ATR-dependent DNA damage signalling cascade. Therefore, although ATM can silence transcription in the vicinity of DSBs occurring in euchromatic regions to prevent chromatin movement and maintain proximity of broken termini [3] , it does not regulate transcription at telomeres. On the other hand, we observe that TRF2 directly suppresses TERRA transcription through its homodimerization domain. The TRFH domain of TRF2 has been implicated in chromatin compaction [41] , [42] and it might be involved in sequestering chromosome termini within the T-loop structure [48] , [49] , which may protect the ends of chromosomes from the DNA damage machinery. When TRF2 is removed, the higher order telomere structures are disrupted and the telomeric chromatin becomes accessible to RNAPII. Moreover, the TRFH domain of TRF2 is required to prevent the activation of ATM and the initial steps in the DDR pathway [44] . This observation together with the evidence that the DDR pathways are not responsible for TERRA accumulation, lead us to hypothesize that TERRA may function either upstream or in parallel to ATM signalling upon telomere deprotection. What is then the role of TERRA upregulation at uncapped telomeres? In addition to its roles in telomere end processing [50] , we propose a functional link between TERRA induction and chromatin reorganization of dysfunctional telomeres. TERRA has been implicated in the accumulation of H3K9me3 at functional telomeres facilitating heterochromatin formation [27] , [29] . Moreover, at elongated telomeres increased density of H3K9me3 correlates with an increase in TERRA-derived UUAGGG signal [27] . Here, we show that the UUAGGG-tract of TERRA interacts with the N-terminal domain of the histone methyltransferase SUV39H1 responsible for the methylation of H3K9. Given that telomeric chromatin requires dynamic remodelling upon DNA damage, the TERRA RNA binding ability of SUV39H1 will likely serve to enhance SUV39H1 telomere association following TRF2 depletion promoting de novo methylation of H3K9. Depletion of SUV39H1 reduced telomere fusion events at TRF2-depleted telomeres indicating that SUV39H1 and possibly accumulation of H3K9me3 are required for efficient end fusions (this study and ref. 46 ). Whether this mechanism involves also activation of Tip60 as seen at canonical DNA DSBs remains to be determined in future experiments. In summary, we provide a comprehensive analysis of the molecular mechanisms underlying TERRA transcriptional regulation at uncapped telomeres and we propose a model in which TERRA acts in the initiation steps of the DDR pathways promoting changes in the chromatin architecture of damaged telomeres and ensuring an effective DDR ( Fig. 8d ). Plasmids shRNA vectors were prepared by cloning double-stranded DNA oligonucleotides into pSuper-Puro or pSuper-Blast. The target sequences were as follows: TRF2, 5′-GCGCATGACAATAAGCAGA-3′ (ref. 50 ); POT1 5′-GTACTAGAAGCCTATCTCA-3′ (shPOT1-2) and 5′-GGGTGGTACAATTGTCAAT-3′ (shPOT1-3) (ref. 51 ); MRE11, 5′-TGAGAACTCTTGGTTTAAC-3′ (ref. 50 ); NBS1, 5′-AGGAAGATGTCAATGTTAG-3′ (ref. 50 ); ATM, 5′-GCAACATACTACTCAAAGA-3′ (ref. 52 ); ATR, 5′- GGAGATTTCCTGAGCATGT-3′ (ref. 53 ); TRF1, 5′-GAATATTTGGTGATCCAAA-3′ (ref. 54 ); hRAP1 5′-AGAGTTCTTGCATTGGAACT-3′ (ref. 55 ); TIN2 5′-GTGGAACATTTTCCGCGAGTACTGGAGT-3′ (ref. 51 ); 5′-GACUUAGAUGUUCAGAAAA-3′ (ref. 51 ); hSMG1a 5′-ATCTTCTGGGAATATTACT-3′ (ref. 23 ); hSMG1b 5′-CACTTCAGATAACTGAGAG-3′ (ref. 23 ). Full-length human TRF1 and TRF2, and chimeric TRF2 constructs were cloned from cDNAs into pCDNA6-based mammalian expression vectors using PCR amplification and InFusion cloning (Clonetech). The full-length SUV39H1 and SUV39H1 deletion mutant cDNA fragments were cloned into bacterial expression plasmids pGEX6p-1. Cell culture and transfection HeLa cells were transfected using Lipofectamine 2000 according to the manufacturer's protocol (Invitrogen). Puromycin (2 μg ml −1 ; InvivoGen) or blasticidin (10 μg ml −1 ; InvivoGen) was added to the medium 24 h after transfection of pSuper-Puro and/or pSuper-Blast constructs. Puromycin and blasticidin selection was maintained for 4 days. siRNA transfections siRNA transfection was performed with Lipofectamine RNAiMAX (Invitrogen, USA) according to the manufacturer’s procedures. SiRNA oligonucleotides sequences were as follows: SUV39H1 siRNAa, 5′-ACCUCUUUGACCUGGACUA-3′ (ref. 56 ), SUV39H1 siRNAb, 5′-CAAAUCGUGUGGUACAGAA-3′ (ref. 57 ), Luciferase siRNA, 5′-CGUACGCGGAAUACUUCGA-3′. Affinity purification of UUAGGG-repeat containing RNA Affinity purification of 5′ capped RNAs was performed by incubating nuclear RNA with GST-eIF4E as described [28] . Briefly, purified GST-eIF4E (1 mg) was bound to glutathione agarose beads in 1 × phosphate-buffered saline (PBS) for 1 h at 4 °C. The beads were washed with 1 × PBS and with buffer A (10 mM KHPO4 pH 8.0, 100 mM KCl, 2 mM EDTA, 5% glycerol, 100 μg ml −1 yeast tRNA, 6 mM DTT, 1.3% polyvinyl alcohol, Triton X-100, 1 U μl −1 SuperaseIN (Ambion)) and then incubated with nuclear RNA, pre-heated to 75 °C for 5 min, at room temperature. After 1 h, the supernatant was collected and the beads were washed five times with 1 ml buffer A lacking yeast tRNA. RNA retained on the beads as well as RNA present in the supernatant fraction was extracted using the RNeasy Mini Kit (Qiagen), according to the manufacturer instructions. A total of 125 μg of nuclear RNA pulled down with GST-eIF4E was then incubated with 125 pmol of (CCCTAA) 3 oligonucleotide in 250 μl of 5 mM Tris–HCl pH 7.5, 0.5 mM EDTA and subsequently heated to 75 °C for 5 min to denature the RNA secondary structures. NaCl was added to a final concentration of 1 M and the sample was cooled down to 50 °C over a period of 30 min. Then, 25 μl of Dynabeads (10 mg ml −1 ; Invitrogen) were added and the mixture was incubated at 50 °C for 3 h. After washing the beads, the RNA was eluted by adding 100 μl of 10 mM Tris–HCl pH 8.0 and heating to 80 °C for 3 min. DSN library preparation and RNA high-throughput sequencing Libraries were prepared starting from 100 ng of RNA using the PE-102-1002-Paired-end kit from Illumina (Illumina, San Diego, CA, USA) according to manufacturer’s recommendations. Ligation products of around 250 bp were gel purified before PCR amplification (15 cycles). Then 100 ng of libraries were normalized according to the Illumina DSN protocol using the Duplex-specific nuclease from Evrogen (JSC, Moscow, Russia). Twelve PCR cycles were performed using PCR PE 1.0 and 2.0 primers to enrich DNA fragments. DSN libraries were loaded on a HiSeq 2000 (Illumina) at 6 pM and paired-end sequenced using the 100 bp protocol. The RNA-seq data sets were submitted to NCBI GEO and have the accession number GSE56727. Mapping RNA-seq to human subtelomeres The sequencing produced 100 nucleotide (nt) paired-end reads from each of the four different samples. FLASH [58] was used to merge overlapping mates into single-end reads. We used FastQC ( http://www.bioinformatics.babraham.ac.uk/projects/fastqc ) for the quality control. After sequencing quality control, the first 10 and the last five bases were trimmed, leaving read lengths of 85 nucleotides. Except for telomere 1p, the reads were subsequently mapped to a set of 500,000 nt-sized subtelomere assemblies (Wistar Institute, http://www.wistar.org/lab/harold-c-riethman-phd/page/subtelomere-assemblies ) with Bowtie [59] (via the HTSstation [60] ). Coordinate 1 of each completed assembly corresponds to the start of the terminal repeat tract on the strand oriented towards the centromere (to maintain a consistent starting coordinate for subtelomere annotation). For the telomeres whose reference sequence does not extend to the terminal repeat (6p, 8p, 11p, 3q, 9q, 20p), coordinate 1 corresponds to the most distal base of the subtelomere assembly. The five acrocentric short-arm telomeres are not represented in these assemblies; while they are known to contain a characteristic SRE organization closely related to distal 4p (ref. 61 ), they cannot be distinguished from each other and assemblies adjacent to them are unavailable. For telomere 1p, the reads were mapped to the subtelomere assembly of NCBI (hg19). Read density profiles were produced counting the number of reads mapping at each position, each read accounting for 1/ N , where N is the number of its different mapping positions. Scores were further normalized by dividing them by the total number of aligned reads for the sample. The ratio plots represent, at each base position within 50 kb from the telomere, the value of one of the ratios in log scale. In cases where the denominator was null, the accounted score was arbitrarily chosen as the log of the numerator. RPKMs of housekeeping genes were calculated using portions of the genome covered by the exons of a given gene (not the whole regions between the Ensembl gene coordinates) as described [33] , whereas RPKM values for TERRA molecules were calculated using the length of each subtelomeric region transcribed into different TERRA species. Northern blot and Real-time RT–PCR Cells were trypsinized and RNA was prepared using the RNeasy Mini Kit (Qiagen), according to the manufacturer’s instructions. For northern blots, RNA (~5 μg) was loaded onto 1.3% formaldehyde agarose gels and separated by electrophoresis. RNA was then transferred to Nylon membranes and blots were blocked in Church buffer for 1 h at 55 °C and then incubated with 32 P-labelled probes. For RT–PCR analysis, total RNA was reverse transcribed with beta-actin [28] and telomere-specific primers ((CCCTAA)5) at 55 °C using SuperScript III reverse transcriptase (Invitrogen). For SYBR green reactions, four different TERRA transcripts were analysed as described previously [28] . Chromatin immunoprecipitation ChIP assays were performed as described previously [51] . For immunoprecipitations, 5 μg of each specific antibody was used, and the mixtures were incubated overnight at 4 °C with 50 μl of a 50% slurry of protein G-Sepharose beads (GE Healthcare). Telomeric DNA was detected with a probe generated as follows: a template mixture of 1–5 kb long telomeric DNA fragments was synthesized by ligating double-stranded telomeric DNA oligonucleotides ((TTAGGG)5, (CCCTAA)5) that were amplified by PCR. The probe was random labelled with α- 32 P-dCTP and cold dTTP and dATP (for detection of the TTAGGG strand). For detection of centromeric sequences, a 5′ 32 P-labelled oligonucleotide probe corresponding to the alphoid element (5′-GTTTTGAAACACTCTTTTTGTAGAATCTGC-3′) was used. RNA-IP RNA-IP of formaldehyde-crosslinked extract was performed as described previously [29] . Briefly, for immunoprecipitations, 5 μg of SUV39H1 or H3K9me3 antibodies were used, and the mixtures were incubated overnight at 4 °C with 50 μl of a 50% slurry of protein G-Sepharose beads (GE Healthcare). TERRA was detected with the telomeric probe as described above. For detection of 18S rRNA, a specific antisense 32 P-γATP 5′-end-labelled oligonucleotide probe was used. Electromobility shift assay EMSA with GST-SUV39H1 was performed in 1 × EMSA reaction buffer (25 mM Tris–HCl pH 8.0, 100 mM NaCl, 10% glycerol, 2 mM MgCl 2 , 1 mM DTT, 1 U μl −1 SuperaseIN). One nanomolar of 32 P-γATP 5′-end-labelled RNA or DNA oligonucleotide probes was mixed with the indicated proteins and competitor oligonucleotides and incubated to equilibrium for 30 min at 37 °C. The reaction was supplemented with EMSA loading buffer to a final concentration of 1 × (8% glycerol, 2 mM Tris-HCl pH 7.5, 0.02% bromophenol blue and cyan cyanol) and separated on 2% 0.5 × TBE-agarose gels at 60 mA for 30 min. Gels were dried, exposed to Phosphoimager screens and analysed using a FLA-3000 Phosphoimager (Fujifilm) and AIDA Image Analyzer software (Raytest). Antibodies The following antibodies were used: Histone H3 (ab1791, Abcam); H3K4me1 (07-436, Millipore); H3K4me2 (07-030, Millipore); H3K4me3 (ab8580, Abcam); H3K9me1 (ab9045, Abcam); H3K9me2 (ab1220, Abcam); H3K9me3 (ab8898, Abcam); SUV39H1#1 (07-958, Millipore); SUV39H1#2 (Active Motif); MRE11 (NB100-142, Novus Biologicals); NBS1 (NB100-143, Novus Biologicals); ATM (Ab-3, Calbiochem); ATR (N19, SantaCruz); phospho-γH2AX (05-636, Millipore), UPF1 (generous gift of Dr. Claus Azzalin) [62] ; α−phospho-(Ser/Thr) ATM/ATR substrate (6966, Cell Signaling). Microscopy IF-FISH staining and telomere-FISH analysis of chromosome metaphase spreads were performed as described [63] . Briefly, for IF-FISH, cover slips were washed with 1 ml 1 × PBS and then fixed with 4% formaldehyde in 1 × PBS for 10 min at room temperature. Subsequently, the cover slips were washed with 1 × PBS, permeabilized in 1 × detergent solution (0.1% Triton X-100, 0.02% SDS in 1 × PBS) and then blocked with 10% normal serum in BSA/1 × PBS. Subsequently, cover slips were incubated with primary and then with secondary antibody, fixed with 4% formaldehyde in 1 × PBS and dehydrated with ethanol. For FISH staining, cover slips were incubated with the hybridization mix, containing 10 mM Tris–HCl pH 7.4, 70% formamide, 0.5% blocking reagent and 1/1,000 Cy3 probe, denatured at 80 °C and hybridized for 3 h at room temperature. After hybridization, cover slips were washed, stained with DAPI and dehydrated with ethanol. For metaphase telomere-FISH, HeLa cells were treated with 0.05 μg Demecolcine for 2 h. Subsequently cells were collected, resuspended in 56 mM KCl at 37 °C for 5 min and then fixed with methanol/acid acetic 3:1 solution. Resuspended cells were dropped onto wet slides, fixed with 4% formaldehyde in 1 × PBS and dehydrated with ethanol. The FISH procedure was performed as described above. Accession codes : The TERRA sequence data have been deposited in NCBI's Gene Expression Omnibus and are accessible through GEO Series accession number GSE56727 ( http://www.ncbi.nlm.nih.gov/geo/query/acc.cgi?acc = GSE56727). How to cite this article: Porro, A. et al. Functional characterization of the TERRA transcriptome at damaged telomeres. Nat. Commun. 5:5379 doi: 10.1038/ncomms6379 (2014).